Earliest known coelacanth skull extends the range of anatomically modern coelacanths to the Early Devonian Coelacanths are known for their evolutionary conservatism, and the body plan seen in Latimeria can be traced to late Middle Devonian Diplocercides , Holopterygius and presumably Euporosteus . However, the group's early history is unclear because of an incomplete fossil record. Until now, the only Early Devonian coelacanth is an isolated dentary ( Eoactinistia ) from Australia, whose position within the coelacanths is unknown. Here we report the earliest known coelacanth skull ( Euporosteus yunnanensis sp. nov.) from the Early Devonian (late Pragian) of Yunnan, China. Resolved by maximum parsimony, maximum likelihood and Bayesian analyses as crownward of Diplocercides or as its sister taxon, the new form extends the chronological range of anatomically modern coelacanths by about 17 Myr. The finding lends support to the possibility that Eoactinistia is also an anatomically modern coelacanth, and provides a more refined reference point for studying the rapid early diversification and subsequent evolutionary conservatism of the coelacanths. Among sarcopterygians (lobe-finned fishes and tetrapods), coelacanths are well known for their evolutionary conservatism [1] , [2] , [3] , in addition to their once prominent role in the study on the origin of tetrapods [1] , [2] , [3] , [4] , [5] . Epitomized by the legendary living fossil Latimeria , the distinctive body plan of anatomically modern coelacanths ( Fig. 1 ) can be traced back to fossil forms from the late Middle Devonian [6] , [7] , [8] , [9] (385.3–391.8 Myr ago; all dates are based on Gradstein et al . [10] ). Many studies have pointed out that coelacanths went through a period of rapid early diversification, but have since displayed remarkable morphological stasis over extended geological time [6] , [7] , [11] , [12] , [13] . A recent study of the HOX clusters of the Indonesian coelacanth Latimeria menadoensis [14] found features indicating stasis in genome evolution that may be correlated with the stasis in morphological evolution. 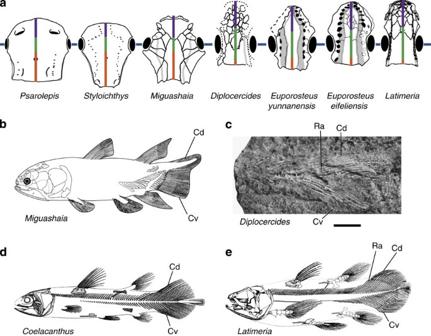Figure 1: Comparison of coelacanth and sarcopterygian body plans. The body plan of anatomically modern coelacanths in comparison to that of primitive coelacanths and non-coelacanth sarcopterygians. (a) Parietonasal or parietal shields from selected sarcopterygians showing different proportions of preorbital, orbital and postorbital regions. Elongated preorbital portion (purple) and orbital portion (green) represent a derived feature characterizingEuporosteusand other anatomically modern coelacanths.Miguashaiaresembles primitive sarcopterygians such asPsarolepisandStyloichthysin having elongated postorbital portion (red). Illustrations modified after referring refs16,19,31. Parietonasal or parietal shields drawn to comparable anteroposterior length and are not to scale. (b–e) Differences in caudal fin between anatomically modern coelacanths and primitive coelacanths.Miguashaia(b) resembles primitive rhipidistians such asGlyptolepisandOsteolepisin having a heterocercal tail.Diplocercides(c),Coelacanthus(d) andLatimeria(e) have a diphycercal or trilobed tail with symmetrically developed dorsal and ventral lobes. Illustrations not to scale;bfrom ref.19;dandefrom ref.7; (c) from ref.20(pl. 6, Fig. 3) with image vertically reversed to show the same anteroposterior orientation asb,d,e. Cd, dorsal lobe of caudal fin; Cv, ventral lobe of caudal fin; Ra, endoskeletal radial. Scale bar, (c) 1 cm. Figure 1: Comparison of coelacanth and sarcopterygian body plans. The body plan of anatomically modern coelacanths in comparison to that of primitive coelacanths and non-coelacanth sarcopterygians. ( a ) Parietonasal or parietal shields from selected sarcopterygians showing different proportions of preorbital, orbital and postorbital regions. Elongated preorbital portion (purple) and orbital portion (green) represent a derived feature characterizing Euporosteus and other anatomically modern coelacanths. Miguashaia resembles primitive sarcopterygians such as Psarolepis and Styloichthys in having elongated postorbital portion (red). Illustrations modified after referring refs 16 , 19 , 31 . Parietonasal or parietal shields drawn to comparable anteroposterior length and are not to scale. ( b – e ) Differences in caudal fin between anatomically modern coelacanths and primitive coelacanths. Miguashaia ( b ) resembles primitive rhipidistians such as Glyptolepis and Osteolepis in having a heterocercal tail. Diplocercides ( c ), Coelacanthus ( d ) and Latimeria ( e ) have a diphycercal or trilobed tail with symmetrically developed dorsal and ventral lobes. Illustrations not to scale; b from ref. 19 ; d and e from ref. 7 ; ( c ) from ref. 20 (pl. 6, Fig. 3) with image vertically reversed to show the same anteroposterior orientation as b , d , e . Cd, dorsal lobe of caudal fin; Cv, ventral lobe of caudal fin; Ra, endoskeletal radial. Scale bar, ( c ) 1 cm. Full size image An important question for studying patterns of the coelacanth evolution is when the anatomically modern coelacanths developed their distinctive body plan. The early fossil record of coelacanths has been scarce, and opinions differ on which sarcopterygian taxon is the closest sister group of coelacanths [15] , [16] . So far, the earliest record of the traditionally defined coelacanth group [3] , [6] , [7] , [17] is one isolated dentary ( Eoactinistia ) from the Early Devonian (late Pragian, ∼ 409 Myr ago) of Australia [17] . Because of its limited morphological features, Eoactinistia cannot be subjected to a phylogenetic analysis and its position within the coelacanths is unknown. Contrary to all expectations for such an early form, Eoactinistia possesses the large dentary sensory pore present in coelacanths from the Carboniferous and younger age, but absent from any of the Middle–Late Devonian forms. The presence of the dentary pore raises the tantalizing possibility that Eoactinistia may be an anatomically modern coelacanth, previously known only from the late Middle Devonian and younger age. However, the unknown phylogenetic position of Eoactinistia and the lack of any other Early Devonian coelacanth fossils make it impossible to weigh this possibility against other possibilities (that is, the dentary pore as an independently derived feature that arose twice among coelacanths, or as a primitive feature that was lost in other Devonian forms but then reappeared in later coelacanths) [17] . Better-known Devonian coelacanths come from the late Middle to early Late Devonian, and had already diverged significantly by that time [7] , [9] , [18] . Gavinia [18] and Miguashaia [19] are considered primitive coelacanths because they resemble primitive lungfishes and porolepiforms and lack features characteristic of the distinctive body plan found in anatomically modern coelacanths. Diplocercides [7] , [20] is positioned crownward of Gavinia and Miguashaia because it possessed the features typical of anatomically modern coelacanths, with two pairs of parietals, an elongated preorbital portion of the skull and a trilobed tail ( Fig. 1 ). Euporosteus was formerly based on one single specimen showing features of the ethmosphenoid and the parietonasal shield [20] , [21] , [22] . It was sometimes left out of phylogenetic analyses because of the limited number of cranial features [7] , [16] , and sometimes placed either crownward of Diplocercides [6] or allied with Diplocercides [7] , [23] . Given its position in reference to Diplocercides , Euporosteus probably belongs to anatomically modern coelacanths even though its postcranial morphology is unknown. Holopterygius is peculiar among the anatomically modern coelacanths in having a specialized eel-like body form. It forms the sister taxon of a Carboniferous coelacanth ( Allenypterus ) and is placed crownward of Diplocercides [9] . In view of 'the probable origin of coelacanths during the Early Devonian or Late Silurian', Friedman and Coates [9] commented on the short interval over which the Devonian forms (for example, Holopterygius and Miguashaia ) developed their morphological distinctness from each other. Although the specialized morphology of Holopterygius from the late Middle Devonian points to the rapid early diversification of coelacanths as a whole, it indirectly raises a similar question as the dentary pore of Eoactinistia , that is, when did the distinctive body plan of the anatomically modern coelacanths first arise, and whether the chronological range of the anatomically modern coelacanths can be extended beyond the late Middle Devonian? Here we report the earliest known coelacanth skull from the Early Devonian (late Pragian) of Zhaotong, Yunnan, China ( Fig. 2 ). Consisting of a parietonasal shield and a postparietal shield, the material resembles Euporosteus eifeliensis from the Middle Devonian of Germany [20] , [21] , [22] and reveals unique features to justify the erection of a new species. In a phylogenetic analysis with new characters added to the data matrix from Friedman and Coates [9] , maximum likelihood and Bayesian analyses place the new form (together with E. eifeliensis ) crownward of Diplocercides . The finding expands the existing knowledge of Euporosteus , and represents the first record of an anatomically modern coelacanth before the late Middle Devonian. The new form extends the chronological range of the anatomically modern coelacanths by about 17 Myr (from the late Middle Devonian to the Early Devonian). It lends support to the possibility that the dentary pore of Eoactinistia may be a synapomorphy indicating its membership among the anatomically modern coelacanths, previously known only from the late Middle Devonian and younger age. It also adds to the growing body of evidence pointing to the South China block as the centre for sarcopterygian diversification [24] , [25] , from which coelacanth representatives were peculiarly absent until now. 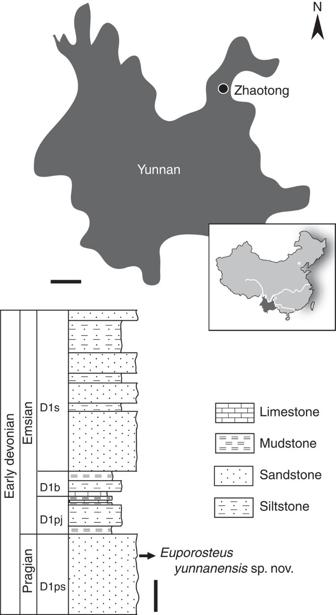Figure 2: Location map and lithocolumn ofEuporosteus yunnanensissp. nov. D1b, Bianqinggou Formation; D1pj, Pojiao Formation; D1ps, Posongchong Formation; D1s, Suotoushan Formation. Scale bar, above, 50 km; below, 50 m. Figure 2: Location map and lithocolumn of Euporosteus yunnanensis sp. nov. D1b, Bianqinggou Formation; D1pj, Pojiao Formation; D1ps, Posongchong Formation; D1s, Suotoushan Formation. Scale bar, above, 50 km; below, 50 m. Full size image Geological setting The new materials were collected in 2009 and 2011 from a yellow sandstone layer of the Posongchong Formation, near Qingmen Reservoir, Zhaotong, Yunnan, China ( Fig. 2 ). In addition to invertebrate lingulids and plants, associated vertebrate faunal members include galeaspid agnathans, placoderms, onychodonts and rhipidistians [26] , [27] . The late Pragian age of the Posongchong Formation is mainly based on the correlation of marine invertebrates and conodonts from the overlying Pojiao Formation yielding the Euryspirifer tonkinensis fauna [28] . Associated plant megafossils (the Posongchong Flora) display obvious endemism, but some cosmopolitan members are shared by the Posongchong Flora and the coeval upper Baragwanathia flora in Australia [29] . Systematic palaeontology Osteichthyes Huxley, 1880 Sarcopterygii Romer, 1955 Actinistia Cope, 1871 Euporosteus Jaekel, 1927 Type species. E. eifeliensis Jaekel, 1927. Distribution. Germany and South China. Emended diagnosis. Elongated preorbital and orbital portions (shared with anatomically modern coelecanths); suturally positioned large pores of the supraorbital sensory canal (shared with anatomically modern coelacanths except for the possibly dimorphic condition in Diplocercides (ref. 20 contra [30] 30)); supraorbital sensory canal wide in diameter, anteriorly converging to meet its counterpart, with a groove marking the path of the inner wall of the canal; surface of dermal bone smooth with no tubercles. Euporosteus yunnanensis sp. nov. Etymology. Specific epithet is from Yunnan, the fossil locality. Holotype. IVPP (Institute of Vertebrate Paleontology and Paleanthropology) V17682.1, a parietonasal shield. Referred material. IVPP V17682.2, a postparietal shield. Locality, horizon and age. Zhaotong, Yunnan Province, China; Posongchong Formation, late Pragian, Early Devonian. Diagnosis. Large supraorbital canal pores in preorbital portion laterally flanked by small pores; preorbital portion anteriorly tapering rather than rounded; postorbital portion of parietonasal shield about one-fifth of total length of the shield; postparietal shield trapezoid in shape, with its maximum width almost equalling its length; posterior margin of the postparietal shield convex, forming pointed protrusions flanking the median embayed area; supratemporal commissure absent from postparietal shield. Description The parietonasal shield (V17682.1), represented by the internal and external moulds, is very similar in overall shape to that of Euporosteus eifeliensis [21] from the late Middle Devonian of Germany. The parietonasal shield is about 11.4 mm long, with its restored maximum width (about 7.8 mm) lying at the level of the preorbital corner ( Fig. 3a–c ). Delimited by the well-developed preorbital and postorbital corners, the preorbital, orbital and postorbital regions, respectively, make up 40%, 41% and 19% of the total length of the shield, approaching the proportions in E. eifeliensis [21] (respectively, 44%, 44% and 12% as judged by the dorsal surface features of the ethmosphenoid). Elongated preorbital and orbital regions represent a derived cranial feature of the anatomically modern coelacanths. In Diplocercides and Latimeria , the respective proportions of the three regions are 42, 51–52 and 6–7% (ref. 31 ). In contrast, respective proportions in Miguashaia [19] are 34, 21 and 45%, similar to those in other primitive sarcopterygians (for example, Psarolepis and Styloichthys ) [15] , [32] , [33] ( Fig. 1a ). 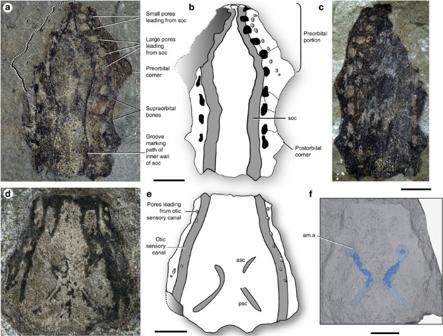Figure 3:Euporosteus yunnanensissp. nov. from the Early Devonian. (a–c) Holotype, IVPP V17682.1, a parietonasal shield. (a) Internal mould. (b) Interpretative drawing. (c) External mould. (d–f) IVPP V17682.2, a postparietal shield in dorsal view, with dermal bones largely eroded. (d) Photo. (e) Interpretative drawing. (f) Computer reconstruction of micro-CT scanning data showing the outline of the semicircular canals by transparency mode. am.a, anterior ampulla; asc, ridge housing anterior semicircular canal; psc, ridge housing posterior semicircular canal; soc, supraorbital sensory canal. Scale bar, 2 mm. Figure 3: Euporosteus yunnanensis sp. nov. from the Early Devonian. ( a – c ) Holotype, IVPP V17682.1, a parietonasal shield. ( a ) Internal mould. ( b ) Interpretative drawing. ( c ) External mould. ( d – f ) IVPP V17682.2, a postparietal shield in dorsal view, with dermal bones largely eroded. ( d ) Photo. ( e ) Interpretative drawing. ( f ) Computer reconstruction of micro-CT scanning data showing the outline of the semicircular canals by transparency mode. am.a, anterior ampulla; asc, ridge housing anterior semicircular canal; psc, ridge housing posterior semicircular canal; soc, supraorbital sensory canal. Scale bar, 2 mm. Full size image The new form resembles anatomically modern coelacanths (except for the possibly dimorphic condition in Diplocercides ; ref. 20 contra [30] 30) in having suturally positioned large pores of the supraorbital sensory canal, and uniquely resembles E. eifeliensis in having a distinct groove marking the path of the inner wall of the wide supraorbital sensory canal. As in E. eifeliensis , a row of about ten very large pores runs antero-posteriorly in the suture line between the lateral and the medial series of bones. Parallel and medial to the row of large pores, a distinct groove marks the path of the inner wall of the wide supraorbital canal. In the preorbital region, this groove converges medially to meet its antimere at an acute angle, in contrast to the condition in E. eifeliensis where the anterior portion of the groove follows a smooth curving path to meet its antimere. As in E. eifeliensis , the actual boundaries between the bones cannot be detected, except for a few short transversely positioned sutures possibly marking the boundaries between some of the bones in the lateral series, such as the supraorbitals ( Fig. 3a,b ). The elongate preorbital portion tapers anteriorly to form a somewhat pointed silhouette, in contrast to the more rounded anterior outline in E. eifeliensis and other coelacanths. Unlike E. eifeliensis , the large sensory pores in the preorbital portion are laterally flanked by a row of small pores, which probably represent the openings for small laterally running branches of the supraorbital sensory canal. No opening for the rostral organ can be distinguished apart from these small pores. The parietonasal shield has a jagged posterior margin, corresponding to the contour presented by the posterior margin of the ethmosphenoid in E. eifeliensis . There are two embayed areas aligned with the grooves marking the supraorbital canal. Lateral to the embayed areas, the posterior margin of the parietonasal shield protrudes posteriorly, roofing over the space that corresponds to the weakly developed descending process of the parietal in E. eifeliensis [21] . The postparietal shield (V17682.2) is about 8.7 mm long and trapezoid in shape ( Fig. 3d–f ). It is narrower anteriorly (about 4.9 mm) and wider posteriorly, with its greatest width (about 8.5 mm) almost equalling its length and lying at the level of the postero-lateral corner of the shield. The ratio between the maximum width and length is 0.98, close to that in some Palaeozoic and Early Triassic coelacanths such as Miguashaia, Diplocercides and Whiteia [19] , [20] , [34] , [35] , [36] . In porolepiforms and many more crownward coelacanths from younger geological age including Latimeria , the postparietal shield is wide and short with the width equalling or exceeding 1.5 times of the length [7] , [31] . The surface of the postparietal shield is smooth and is not ornamented with tubercles, a dermal bone condition also seen in the parietonasal shield of E. efieliensis [20] . The postparietal shield matches the parietonasal shield in terms of proportional size, overall anterior contour, transverse curvature, position of the sensory canals and general preservational condition. However, as the postparietal and parietonasal shields belong to separate individuals, the contours of the respective anterior and posterior margins do not match precisely. The anterior margin of the postparietal shield is not straight, with two tapered anterior protrusions carrying the otic sensory canals that appear to be aligned with the embayed areas in the posterior margin of the parietonasal shield where the supraorbital sensory canals exit the parietonasal shield. A faint stripe marking the otic sensory canal runs longitudinally throughout the postparietal shield, roughly parallel to the lateral margin of the shield. About six to seven small pores lie laterally to the otic sensory canal, resembling the small pores in the preorbital region of the parietonasal shield. Posteriorly, no supratemporal commissure is found branching off from the otic sensory canal, as distinct from the condition in forms such as Coelacanthus [37] and Latimeria [38] , where the supratemporal commissure joins the otic canal in the supratemporal. As the posterior right portion of the postparietal shield is well preserved, the absence of the supratemporal commissure is not due to the preservational condition. The medial branch of the otic sensory canal, and the middle and posterior pit lines are not visible because of poor preservation. The preservational condition also makes it difficult to make out the sutures, and therefore the number of bones forming the lateral margin of the shield cannot be determined. Along the midline in the posterior half of the postparietal shield, two sets of discoloured markings, like the faint stripes marking the otic sensory canals, together present an X-shaped pattern. These paired markings lie close to each other near the midline, resembling the position of the ridges for semicircular canals in the actinopterygian Kansasiella [31] , [39] . As shown by microcomputed tomography (micro-CT) reconstructions, these markings indicate the position of the ridges housing the anterior and posterior semicircular canals ( Figs 3f and 4 ). The reconstructed labyrinth structures appear to be similar to those in Diplocercides , except for the smaller distance between the left and right sets of semicircular canals. 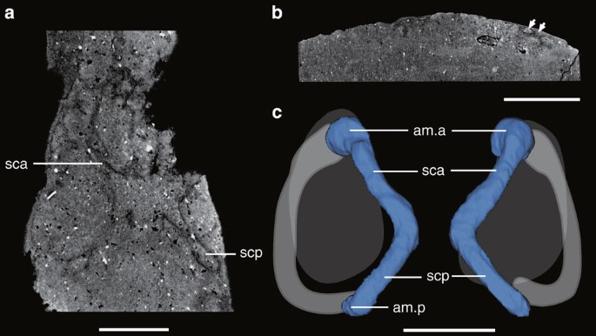Figure 4: Micro-CT images and reconstruction. Micro-CT images and reconstruction showing preserved labyrinth structures ofEuporosteus yunnanensissp. nov. (a) Selected horizontal micro-CT slice showing the anterior and posterior semicircular canals. (b) Selected transverse micro-CT slice through the anterior semicircular canal (arrow). (c) Computer reconstruction of the preserved labyrinth structures (blue) in dorsal view. am.a, anterior ampulla; am.p, posterior ampulla; sca, anterior semicircular canal; scp, posterior semicircular canal. Scale bar, 2 mm. Figure 4: Micro-CT images and reconstruction. Micro-CT images and reconstruction showing preserved labyrinth structures of Euporosteus yunnanensis sp. nov. ( a ) Selected horizontal micro-CT slice showing the anterior and posterior semicircular canals. ( b ) Selected transverse micro-CT slice through the anterior semicircular canal (arrow). ( c ) Computer reconstruction of the preserved labyrinth structures (blue) in dorsal view. am.a, anterior ampulla; am.p, posterior ampulla; sca, anterior semicircular canal; scp, posterior semicircular canal. Scale bar, 2 mm. Full size image The lateral portion of the posterior margin of the postparietal shield tapers posteromedially, ending in two pointed protrusions on either side of the roundish median embayment for the median extrascapular. The phylogenetic position of Euporosteus is critical for deciding whether it represents an anatomically modern coelacanth crownward of (or at least not basal to) Diplocercides , which is known to have postcranial anatomy [20] similar to stratigraphically younger and phylogenetically more crownward coelacanths, including the modern coelacanth Latimeria ( Fig. 1 ). Because of the limited number of cranial features seen in E. eifeliensis , inclusion of the previously monotypic Euporosteus in cladistic analyses tended to increase the number of resulting trees or cause the collapse of many basal coelacanths crownward of Miguashaia [7] . Cloutier [6] placed Euporosteus crownward of Diplocercides presumably because of the possession of large pores for the sensory canal places, but this feature must now be regarded as dimorphic in Diplocercides because a recently reported Diplocercides skull from Gogo also has large sensory canal pores [30] . Forey [7] included Euporosteus in the original data matrix with 30 coelacanth genera as the ingroup, but it was later removed from the analysis, together with 5 other genera with many missing values. After conducting a re-weighted analysis with the truncated data set, Forey [7] obtained one single tree with 24 coelacanth taxa. Forey then added the six previously removed genera 'at nodes or along branches commensurate with their real data' and Euporosteus was placed on the same branch as Diplocercides . Friedman and Coates [9] expanded Forey's data matrix by adding Holopterygius , and removed the same six genera (including Euporosteus ) from the analysis. Using a data matrix with 39 taxa (5 of which are members of the traditionally recognized coelacanths) and 159 characters, Friedman [16] found that Euporosteus 'wanders freely within the coelacanth clade' and pruned Euporosteus from the constituent trees before producing a reduced-consensus topology. To explore the phylogenetic position of Euporosteus in the light of the new material, an expanded data matrix of 29 taxa and 115 morphological characters is assembled based on Friedman and Coates [9] and Forey [7] . Gavinia [18] and six new characters (Characters 110–115) are added to the data matrix ( Supplementary Methods and Supplementary Note 1–3 ). The codings of Euporosteus are derived from the data set of Forey [7] and amended from features revealed by the postparietal shield of E . yunnanensis , such as the absence of the supratemporal commissure on the postparietal shield (Character 21), and the width/length ratio of the postparietal shield (Character 115). The codings for other taxa, including those of Actinopterygii and Porolepiformes as outgroups, follow Forey [7] as modified in Friedman and Coates [9] . Although the results resemble previous analyses in revealing many problematic areas of the coelacanth phylogeny requiring future studies, the position of Euporosteus (either crownward of Diplocercides or as its sister taxon) gains more explicit support than in previous analyses. Euporosteus is placed crownward of Diplocercides in the Bayesian and randomized axelerated maximum likelihood (RaxML) trees ( Fig. 5 ), as well as in the 50% majority-rule consensus tree ( Supplementary Fig. S1a ) of the 220 shortest trees produced by the maximum parsimony analysis ( Supplementary Methods and Supplementary Note 1–3 ). A re-weighted analysis of the data matrix based on the re-scaled consistency indices of characters places Euporosteus as the sister taxon of Diplocercides ( Supplementary Fig. S2 ), corroborating some of the previous groupings [7] , [23] . However, the strict consensus tree of the 220 shortest trees ( Fig. 5a ) still places Diplocercides , Euporosteus and other anatomically modern coelacanths in a polytomous clade crownward of Miguashaia and Gavinia . 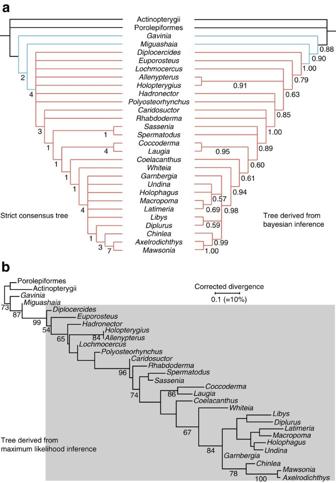Figure 5: Phylogenetic placement ofEuporosteus. (a) The tree derived from Bayesian inference (right) placesEuporosteuscrownward ofDiplocercides. The strict consensus tree of the 220 shortest trees (left) placesDiplocercides,Euporosteusand other anatomically modern coelacanths in a polytomy crownward ofMiguashaiaandGavinia(tree length: 261 steps; consistency index: 0.46; retention index: 0.71; re-scaled consistency index: 0.33). Bremer support values are shown at nodes. (b) Maximum likelihood inference placesEuporosteuscrownward ofDiplocercides. The node for the anatomically modern coelacanths, includingEuporosteusandDiplocercides, is supported by likelihood bootstrap value of 99%. Anatomically modern coelacanths in grey highlight area. Figure 5: Phylogenetic placement of Euporosteus . ( a ) The tree derived from Bayesian inference (right) places Euporosteus crownward of Diplocercides . The strict consensus tree of the 220 shortest trees (left) places Diplocercides , Euporosteus and other anatomically modern coelacanths in a polytomy crownward of Miguashaia and Gavinia (tree length: 261 steps; consistency index: 0.46; retention index: 0.71; re-scaled consistency index: 0.33). Bremer support values are shown at nodes. ( b ) Maximum likelihood inference places Euporosteus crownward of Diplocercides . The node for the anatomically modern coelacanths, including Euporosteus and Diplocercides , is supported by likelihood bootstrap value of 99%. Anatomically modern coelacanths in grey highlight area. Full size image Based on the phylogenetic position of Euporosteus (either crownward of Diplocercides or as its sister taxon), it is parsimonious to predict that Euporosteus should possess the trilobed tail seen in Diplocercides and other anatomically modern coelacanths. Although the absence of postcranial materials calls for proper caution regarding this prediction, the possibility that Euporosteus might have primitive postcranial features is very low (though not inconceivable) because all the coelacanths known so far fall on either side of the morphological gap between primitive forms and anatomically modern forms [7] , and no intermediate or 'chimera' forms have been found. The finding of the earliest coelacanth skull has wide implications for studying the early diversification and paleogeographic distribution of the coelacanths. E . yunnanensis extends by 17 Myr the chronological range of Euporosteus . As the earliest anatomically modern coelacanth, it shows that the distinctive body plan seen in the living fossil Latimeria has remained basically unchanged from the Early Devonian to modern time ( Fig. 6 ). E . yunnanensis lends support to the possibility that Eoactinistia may represent an early member of the anatomically modern coelacanths with the dentary sensory pore. The new form fills in the previously puzzling absence of coelacanth representatives from the Early Devonian of the South China block, which has yielded early members of all other groups of sarcopterygian fishes and is regarded as the centre of origin and diversification of early sarcopterygians. Together with recent findings of onychodonts ( Bukkanodus and Qingmenodus ) [26] , [40] , the distribution of early coelacanths ( Eoactinistia and Euporosteus ) from the Pragian of Australia and South China also suggests the Pragian biogeographic proximity between East Gondwana and the South China block. The finding bodes well for future coelacanth discoveries from the Pragian and earlier strata, and makes the early rapid acquisition of coelacanth characters and the subsequent evolutionary conservatism more impressive than previously thought. 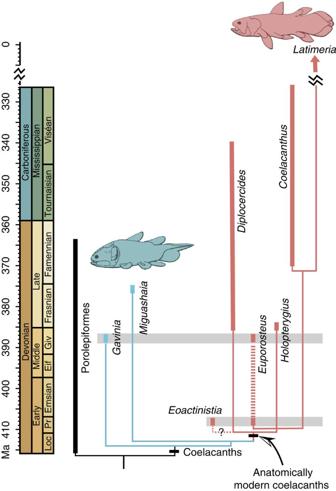Figure 6: Relationship and geological time range of representative coelacanths and related forms. Primitive coelacanths are in light blue and the anatomically modern coelacanths including extantLatimeriaare in red.Euporosteusis positioned either crownward ofDiplocercidesor as its sister taxon, indicating that the distinctive body plan of anatomically modern coelacanths must have been established no later than 409 million years ago (Ma).Euporosteusalso lends support to the possibility thatEoactinistiamay represent an early member of the anatomically modern coelacanths with the dentary sensory pore. Eif, Eifelian; Giv, Givetian; Loc, Lochkovian; Pr, Pragian. Figure 6: Relationship and geological time range of representative coelacanths and related forms. Primitive coelacanths are in light blue and the anatomically modern coelacanths including extant Latimeria are in red. Euporosteus is positioned either crownward of Diplocercides or as its sister taxon, indicating that the distinctive body plan of anatomically modern coelacanths must have been established no later than 409 million years ago (Ma). Euporosteus also lends support to the possibility that Eoactinistia may represent an early member of the anatomically modern coelacanths with the dentary sensory pore. Eif, Eifelian; Giv, Givetian; Loc, Lochkovian; Pr, Pragian. Full size image Phylogenetic analysis The character data entry and formatting were performed in Mesquite (version 2.5) [41] . All characters were treated as unordered and weighted equally. The data matrix was subjected to the parsimony analysis in PAUP* (version 4.0b10) [42] . Tree searches were conducted using the heuristic algorithm, with 'simple' sequence replicates and 'maxtrees' set to 'automatically increase'. The characters were also re-weighted by their re-scaled consistency indices in a subsequent re-analysis. MacClade 4.0 (ref. 43 ) was used to trace the character transformation in the selected cladogram. Bremer decay indices were obtained using command files composed by TreeRot [44] in conjunction with the heuristic search algorithm in PAUP*. Bayesian inference analyses were conducted using MrBayes 3.1.2 (refs 45 , 46 ). Actinopterygians were set as the outgroup, and the coding showing polymorphisms were changed to '?'. Priors were kept at their default settings for standard (=morphological) analyses. The analysis was run for 1×10 6 generations. Samples were taken every 1×10 2 generations, resulting in a total of 1×10 4 samples for each of the parallel analyses. The first 2.5×10 3 samples for each run, representing the 'burn-in' period, were discarded. The 50% majority-rule consensus tree was computed for the sampled generations ( Fig. 5a , right). The maximum likelihood (RaxML) analyses ( Fig. 5b ) were conducted using RAXML v.7.2.8 (ref. 47 ), with 1,000 bootstraps followed by a maximum likelihood search. Commands used were '-f a -m MULTIGAMMA -K MK -#1,000'. The 50% majority-rule consensus tree was computed for the 1,000 bootstrap trees. Both likelihood-based analyses (Bayesian inference and RaxML) used the stochastic model [48] with a γ -parameter to account for rate variation across traits. The maximum parsimony analysis produced 220 most parsimonious trees of 261 steps (consistency index=0.4598; homoplasy index=0.5402; retention index=0.7122; re-scaled consistency index=0.3275). The strict consensus tree of 220 shortest trees ( Fig. 5a , left) places Gavinia and Miguashaia basal to Diplocercides on the coelacanth lineage. Euporosteus, Diplocercides, Hadronector , Lochmocercus , Polyosteorhynchus, Holopterygius and Allenypterus appear in a polytomy with the less inclusive clade ( Caridosuctor + Rhabdoderma +all more crownward coelacanths). In the 50% majority-rule consensus tree ( Supplementary Fig. S1a ), Euporosteus is placed as a sister taxon of Holophagus and Allenypterus , crownward of Diplocercides . The analysis with characters reweighted by their re-scaled consistency indices results in two shortest cladograms (tree length=86.1112; consistency index=0.7031; homoplasy index=0.2969; retention index=0.8861; re-scaled consistency index=0.6230), both placing Euporosteus as the sister taxon of Diplocercides ( Supplementary Fig. S2 ). The maximum likelihood and Bayesian inferences produced almost consistent results although the maximum likelihood tree is less resolved in several nodes than the Bayesian tree. The trees based on maximum likelihood and Bayesian methods have an overall topology similar to the most parsimonious trees, but some differences still exist. As in the 50% majority-rule consensus tree, the Bayesian and maximum likelihood inferences place Euporosteus crownward of Diplocercides , and the grouping of Holophagus and Allenypterus is well recognized. However, in the Bayesian analyses, Hadronector and Polyosteorhynchus are placed in a polytomy with the less inclusive clade ( Caridosuctor +all more crownward coelacanths), representing a departure from the consensus tree based on the maximum parsimony. X-ray micro-CT The X-ray micro-CT scan was carried out using the 225KV micro-CT (developed by the Institute of High Energy Physics, CAS) at the Key Laboratory of Evolutionary Systematics of Vertebrates, Chinese Academy of Sciences (CAS). The specimen was scanned with beam energy of 130 kV and a flux of 90 μA at a detector resolution of 10.8 μm per pixel using a 720° rotation with a step size of 0.5° and an unfiltered aluminium reflection target. A total of 1,440 transmission images were reconstructed in a 2,048×2,048 matrix of 1,563 slices in a two-dimensional reconstruction software developed by the Institute of High Energy Physics, CAS. The three-dimensional reconstructions were created in the software Mimics (version 14.12), and images of the reconstructions were exported from Mimics and finalized in Adobe Photoshop and Adobe Illustrator. How to cite this article: Zhu, M. et al . Earliest known coelacanth skull extends the range of anatomically modern coelacanths to the Early Devonian. Nat. Commun. 3:772 doi: 10.1038/ncomms1764 (2012).